IMGT/HighV QUEST paradigm for T cell receptor IMGT clonotype diversity and next generation repertoire immunoprofiling T cell repertoire diversity and clonotype follow-up in vaccination, cancer, infectious and immune diseases represent a major challenge owing to the enormous complexity of the data generated. Here we describe a next generation methodology, which combines 5′RACE PCR, 454 sequencing and, for analysis, IMGT, the international ImMunoGeneTics information system (IMGT), IMGT/HighV-QUEST web portal and IMGT-ONTOLOGY concepts. The approach is validated in a human case study of T cell receptor beta (TRB) repertoire, by chronologically tracking the effects of influenza vaccination on conventional and regulatory T cell subpopulations. The IMGT/HighV-QUEST paradigm defines standards for genotype/haplotype analysis and characterization of IMGT clonotypes for clonal diversity and expression and achieves a degree of resolution for next generation sequencing verifiable by the user at the sequence level, while providing a normalized reference immunoprofile for human TRB. The T cell receptor (TR) [1] is critical for peptide/major histocompatibility (pMH) recognition. The TR repertoire is vast, with direct estimates of 2.5 × 10 7 unique αβ TR per individual [2] and significantly higher numbers by theoretical calculations [3] . The αβ TR is a membrane-bound, clonotypic, heterodimeric protein comprising one alpha chain (TRA) and one beta chain (TRB) [1] . Each chain comprises a variable (V) domain and a constant (C) region that includes a C domain and connecting, transmembrane and cytoplasmic regions. The V-ALPHA domain results from the rearrangement between a TRAV gene and a joining J ( TRAJ ) gene, whereas the V-BETA domain results from the rearrangement of a TRBV gene, a diversity D ( TRBD ) gene and a joining J ( TRBJ ) gene. The C region of the TR chains is encoded by the TRAC and TRBC ( TRBC1 and TRBC2 ) genes, respectively [1] . Each V domain comprises three highly flexible complementarity-determining regions (CDR) at the antigen-binding face of the receptor [1] . When docking its cognate pMH ligand, the CDR1 and CDR2 facilitate binding of the receptor to the MH helices, while CDR3 principally engages the peptide within the MH groove [4] , [5] . The specificity of the TR predominantly depends on the CDR3 created by the V-(D)-J rearrangement. It remains a significant challenge to understand the diversity and specificity of T cells, particularly during natural infection. The approach by tetramer staining or antigen-induced cytokine release [6] , [7] , [8] , [9] , [10] , [11] is limited by our knowledge of mapped epitopes. Classical DNA cloning and Sanger sequencing techniques are laborious and generally limit data to a few hundred, or in rare cases a few thousand, TR sequences per investigation [6] , [7] , [8] , [9] . The complexity and depth of the human TR repertoire was recently explored in several studies using next generation sequencing (NGS) [12] , [13] , [14] , [15] , [16] , [17] , [18] , [19] , [20] . In these studies, Illumina sequencing was primarily used, with a major advantage of generating very deep data, but a disadvantage that the read length was short and the data either required assembly [12] , [13] or focused exclusively on the CDR3 (refs 14 , 15 ). 454 sequencing was also used previously [16] , [17] , [19] , [20] but only in combination with multiplex PCR. Earlier studies also explored various bioinformatic tools but different algorithms added potential layers of discrepancy. ImMunoGeneTics (IMGT)/HighV-QUEST [21] , [22] ( http://www.imgt.org ) is the authentic high throughput version of the IMGT/V-QUEST tool [23] , [24] , [25] (acknowledged as the international reference for immunoglobulin and TR sequence analysis, CSH Protocols, WHO/IUIS). IMGT/HighV-QUEST uses the same algorithm as IMGT/V-QUEST and achieves the same degree of resolution and high quality results. We now introduce a high throughput methodology for a standardized comparative TR analysis on the basis of IMGT-ONTOLOGY concepts. This approach consists of 5′ rapid amplification of cDNA ends (RACE) [12] , [26] to avoid amplification bias associated with multiplex PCR, 454 sequencing to bypass the limitations of short-read assembly and IMGT/HighV-QUEST analysis [21] , [22] to ensure the highest quality in sequence interpretation of full-length rearranged human TR V-BETA transcripts. We illustrate the usefulness and application of this methodology by the analysis of the human TR repertoire response towards a model immune challenge, the H1N1 vaccine. IMGT/HighV-QUEST was recently released [21] , and this report represents its official initial reference for application in high throughput TR repertoire and IMGT clonotype analysis. Workflow results A model immune challenge was provided by vaccinating a healthy volunteer with a H1N1 influenza vaccine. Three T cell subpopulations (‘CD4 −’ , ‘CD4 +’ and ‘Treg’ [27] , [28] , [29] , [30] ) were isolated by flow cytometry, at four time points (baseline and days 3, 8 and 26 post vaccination) ( Fig. 1a ). Twelve amplicon libraries of the corresponding TR trancripts were prepared using anchored 5′RACE PCR [12] and a TRBC gene-specific reverse primer [1] , [31] ( Supplementary Table S1 ). Sequencing was performed using 454 technology, which is appropriate for >400 nt long sequences. During the platform-specific data processing, 160,944 reads passed the 454 pipeline filter (the pass rate was 46.73%), but 7,405 of these were later discarded owing to missing or incomplete barcodes. Therefore, we obtained 153,539 ‘final 454-output’ reads for the 12 samples, of which 72% exceeded 300 nt. These reads were directly analysed by IMGT/HighV-QUEST, without the need for computational read assembly. 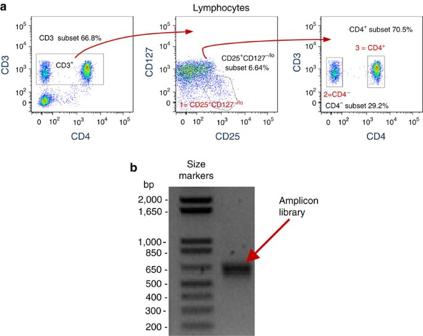Figure 1: Flow cytometry and generation of the final amplicon library. (a) Sorting gate. The initial gates were set on lymphocytes based on side scatter (SSC) and forward scatter (FSC), from which the CD3 T cell gate (left panel) was set. Within the CD3 gate, we firstly gated for CD3+CD25+CD127−/lonatural Treg (‘Treg’) cell population (middle panel) and the remaining CD3+T cells were divided into CD3+CD4+(‘CD4+’) and CD3+CD4−(‘CD4−’) conventional T cells (right panel). (b) Gel appearance of the final purified amplicon library. RNA was purified from sorted cells representing the 12 samples (corresponding to three T cell subpopulations at the four time points) and TRB V-D-J transcripts were amplified, independently, through 5′RACE and PCR and barcodes incorporated in a second PCR. The products were purified and an equal amount (100 ng) of cDNA from each of the 12 reactions was pooled. The final amplicon library appeared as a band between 550 and 650 bp. Figure 1: Flow cytometry and generation of the final amplicon library. ( a ) Sorting gate. The initial gates were set on lymphocytes based on side scatter (SSC) and forward scatter (FSC), from which the CD3 T cell gate (left panel) was set. Within the CD3 gate, we firstly gated for CD3 + CD25 + CD127 −/lo natural Treg (‘Treg’) cell population (middle panel) and the remaining CD3 + T cells were divided into CD3 + CD4 + (‘CD4 +’ ) and CD3 + CD4 − (‘CD4 − ’) conventional T cells (right panel). ( b ) Gel appearance of the final purified amplicon library. RNA was purified from sorted cells representing the 12 samples (corresponding to three T cell subpopulations at the four time points) and TRB V-D-J transcripts were amplified, independently, through 5′RACE and PCR and barcodes incorporated in a second PCR. The products were purified and an equal amount (100 ng) of cDNA from each of the 12 reactions was pooled. The final amplicon library appeared as a band between 550 and 650 bp. Full size image As IMGT/HighV-QUEST currently accepts up to 150,000 sequences per job, the final 454-output 5′ reads (79,564 ‘MIDA_all’) and 3′ reads (73,975 ‘MIDB_all’) were submitted separately ( Supplementary Fig. S1 ). Online statistical analyses (IMGT/HighV-QUEST currently accepts up to 450,000 results of analysed sequences per statistical run) were performed on the pooled results of the two jobs ‘MIDA_all’ and ‘MIDB_all’, and on the combined 5′+3′ reads of each of the 12 samples (designated as sets, for example, MID1 ( Supplementary Table S1 )). An additional level of expertise was specifically developed during this study to define and characterize individual IMGT clonotypes unambiguously from NGS data (clonal diversity) and determine the precise number of sequences assigned to each clonotype (clonal expression). This approach is on the basis of IMGT-ONTOLOGY [32] , [33] and more specifically on the concepts of classification (gene and allele nomenclature) [34] , description (standardized labels) [35] and numerotation (IMGT unique numbering) [36] , [37] , [38] . IMGT/HighV-QUEST summary The IMGT/HighV-QUEST ‘Summary’ of the statistical analysis ( Fig. 2 ) made on ‘MIDA+MIDB’ (pooled results of the two jobs ‘MIDA_all’ and ‘MIDB_all’) shows that, of the 153,539 submitted sequences, 63,371 were categorized as ‘1 copy’ and 867 were categorized as ‘More than 1’. These sequences were filtered-in for statistical analysis (64,238 sequences, 41.84% of the submitted sequences), whereas sequences not answering the required criteria (e.g., ‘No results’, ‘Unknown functionality’) were filtered out [21] ( Supplementary Fig. S1 ). The ‘1 copy’ category (63,371, 98.65% of the filtered-in sequences) comprises the sequences to be analysed in detail (this category avoids repeating the same analysis on strictly identical sequences, which are stored instead in ‘More than 1’) ( Supplementary Fig. S1 ). NGS ‘1 copy’ is not synonymous of ‘clonotype’: indeed, several ‘1 copy’ sequences may correspond to a single clonotype if the sequences only differ in their length and/or due to sequencing errors. One of the aims of this work was therefore to define, identify and characterize the distinct clonotypes from this ‘1 copy’ category, and thus to be able to evaluate the true clonal diversity. 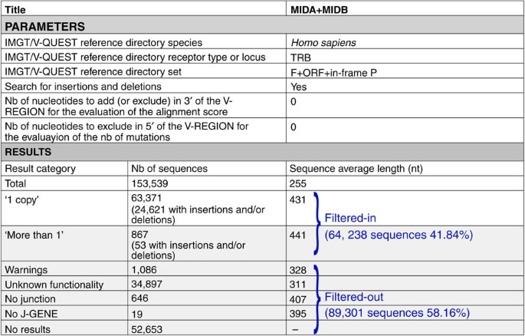Figure 2: IMGT/HighV-QUEST summary. This figure represents a screenshot from IMGT/HighV-QUEST online. The 153,539 sequences ‘MIDA+MIDB’ submitted for detailed statistical analysis correspond to the pooled results of the IMGT/HighV-QUEST jobs 5′ reads ‘MIDA_all’ and 3′ reads ‘MIDB_all’. Parameters used for these analyses are recalled in the top of the IMGT/HighV-QUEST ‘Summary’ table. The lower part of the table shows the classification of the sequences in the ‘Results category’21. Figure 2: IMGT/HighV-QUEST summary. This figure represents a screenshot from IMGT/HighV-QUEST online. The 153,539 sequences ‘MIDA+MIDB’ submitted for detailed statistical analysis correspond to the pooled results of the IMGT/HighV-QUEST jobs 5′ reads ‘MIDA_all’ and 3′ reads ‘MIDB_all’. Parameters used for these analyses are recalled in the top of the IMGT/HighV-QUEST ‘Summary’ table. The lower part of the table shows the classification of the sequences in the ‘Results category’ [21] . Full size image IMGT/HighV-QUEST is a generic tool, and the ‘More than 1’ category is designed for expression studies, in experiments with well-controlled parameters. Indeed, for each ‘1 copy’ sequence, the tool provides the number of ‘More than 1’ sequences (867 sequences, Fig. 2 ; Supplementary Fig. S1 ). A second aim of this work was therefore to assign, to each distinct clonotype, all the relevant ‘1 copy’ sequences, as well as the number of their corresponding ‘More than 1’, and thus to be able to provide the framework to evaluate the clonal expression. IMGT/HighV-QUEST detailed statistical analysis is performed on the ‘1 copy’ sequences. These sequences have an average length of 431 nt ( Fig. 2 ) but the length of the V domain (V-D-J-REGION) within each sequence may vary. With the longer V-D-J-REGION, IMGT/HighV-QUEST identifies a single allele, unambiguously, whereas with the shorter V-D-J-REGION, the tool proposes several solutions. The ‘1 copy’ therefore comprises two categories: ‘single allele’ (one allele for V and J) and ‘several alleles (or genes)’ (several alleles for V and/or J) ( Supplementary Fig. S1 ). In this study, the ‘single allele’ (for V and J) comprised 58,958 sequences (91.78% of the filtered-in sequences, average length 440 nt), with a V-D-J-REGION average length of 335 nt, whereas the ‘several alleles (or genes)’ (for V and/or J) comprised 4,413 sequences (6.87% of the filtered-in sequences, average length 309 nt) with a V-D-J-REGION average length of ~250 nt. Most of the ‘single allele’ sequences contained a complete V domain, with many even containing the leader region (L-REGION) or part of it (checked with the individual sequence files). We consider the sequences of the ‘single allele’ category to be superior to those of the ‘several alleles (or genes)’ category in terms of biological interpretations. IMGT/HighV-QUEST analysis is performed by default with the option of accepting insertions and/or deletions (indels) that looks for indels in the V-REGION and corrects these before characterizing the sequences [22] , [25] . More than 38% (38.41%) of the filtered-in sequences (24,674 sequences out of 64,238, Fig. 2 ) were detected by IMGT/HighV-QUEST as having indels. Most, if not all, of these indels correspond to sequencing errors and therefore the corresponding sequences corrected by IMGT/HighV-QUEST could be included in the final results, as they had no other anomaly. The IMGT/HighV-QUEST option of accepting insertions and/or deletions is therefore particularly appropriate for the 454 sequencing of TR. Analysis without that option would have led these sequences being assigned to one of the filtered-out categories or to an erroneous sequence characterization. TRB genotype and haplotype identification The TRBV , TRBD and TRBJ gene and allele usage was obtained using the statistical analysis of IMGT/HighV-QUEST available online [21] . This analysis is performed automatically on the ‘1 copy’ ‘single allele’ (for V and J) category ( Supplementary Fig. S1 ). A total of 55 TRBV genes (47 functional F, 1F/open reading frame (ORF), 3 ORF, 4 pseudogenes) were identified in the rearrangements. This includes the TRBV6-3 gene as discussed below. The presence of rearranged transcripts for four in-frame pseudogenes TRBV1 , TRBV3-2 , TRBV12-1 and TRBV21-1 was rather unexpected ( Fig. 3a ), but consistent with the selection of the IMGT/V-QUEST directory ‘F+ORF+in-frame P’ for the analysis ( Fig. 2 ). These pseudogenes were found with in-frame or out-of-frame junction rearrangements. Although a limited number of ‘1 copy’ ‘single allele’ for two of these pseudogenes was observed (three for TRBV1 and two for TRBV12-1; Fig. 3a ), the fact that they were found in different sets with different junctions underline the quality of the data and confirmed that no TRBV gene was overlooked in the 5′RACE amplification step. The TRBV3-2 and TRBV21-1 in-frame pseudogenes were found in 105 sequences (56 for allele TRBV3-2*01 and 49 for allele TRBV3-2*03) and 549 sequences, respectively ( Fig. 3a ). In contrast, two other in-frame pseudogenes ( TRBV12-2 and TRBV26 ) and two ORF (TRBV7-1 and TRBV17) were not found ( Fig. 3a ). 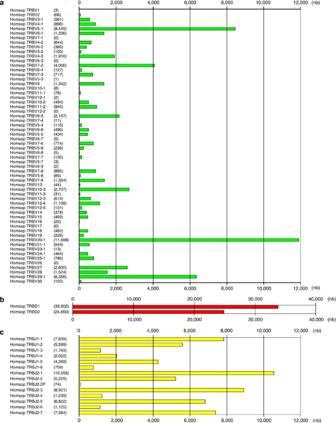Figure 3:TRBgene usage for genotype analysis. Histograms for theTRBVgenes (a),TRBDgenes (b) andTRBJgenes (c) display results from the ‘1 copy’ ‘single allele’ (for V and J) (58,958 sequences, average sequence length of 440 nt, average V-D-J-REGION length of 335 nt), which are the result output from the IMGT/HighV-QUEST detailed statistical analysis performed on ‘MIDA+MIDB’. The histograms show the genes, per group, from 5′ to 3′ in the TRB locus1, with the number of sequences shown in parentheses. TheTRBV30gene is located downstream of theTRBC2gene in the opposite orientation of transcription1. TRBD1 is upstream of TRBJ1-1 and TRBD2 upstream of TRBJ2-1 (ref.1). The histograms of theTRBDandTRBJgenes are displayed separately, owing to the differences of scale (sequences being assigned to 2 and 13 genes, respectively). These histograms and corresponding tables online allow a genotype and haplotype identification if the sequences are obtained from a single individual, as in this study. They include rearranged sequences with in-frame and out-of-frame junctions. Figure 3: TRB gene usage for genotype analysis. Histograms for the TRBV genes ( a ), TRBD genes ( b ) and TRBJ genes ( c ) display results from the ‘1 copy’ ‘single allele’ (for V and J) (58,958 sequences, average sequence length of 440 nt, average V-D-J-REGION length of 335 nt), which are the result output from the IMGT/HighV-QUEST detailed statistical analysis performed on ‘MIDA+MIDB’. The histograms show the genes, per group, from 5′ to 3′ in the TRB locus [1] , with the number of sequences shown in parentheses. The TRBV30 gene is located downstream of the TRBC2 gene in the opposite orientation of transcription [1] . TRBD1 is upstream of TRBJ1-1 and TRBD2 upstream of TRBJ2-1 (ref. 1 ). The histograms of the TRBD and TRBJ genes are displayed separately, owing to the differences of scale (sequences being assigned to 2 and 13 genes, respectively). These histograms and corresponding tables online allow a genotype and haplotype identification if the sequences are obtained from a single individual, as in this study. They include rearranged sequences with in-frame and out-of-frame junctions. Full size image For the first time, the TRBV genotype and haplotypes of an individual could be identified unambiguously from the gene and allele usage ( Supplementary Table S2 ). The apparent ‘absence’ of the functional TRBV6-3 gene was expected as its allele TRBV6-3*01 has an identical sequence to TRBV6-2*01 (the IMGT/HighV-QUEST ‘1 copy’ results therefore include TRBV6-3*01 under ‘TRBV6-2*01). The TRBV6-3 gene was taken into account in the genotype identification ( Supplementary Table S2 ), although it cannot be displayed in the histogram ( Fig. 3a ). No other similar case was detected. The individual is homozygous for most functional TRBV genes, except for 2, for which he is heterozygous, namely TRBV20-1 (alleles *01 and *02) and TRBV7-3 (allele *01 functional and allele *02 ORF). The TRBV genes for which the individual is homozygous have the allele *01, except for three genes, which have the allele *02 (TRBV5-5*02, TRBV15*02 and TRBV30*02). The frequently used V genes are distributed along the TR locus at uneven intervals ( Fig. 3a ). The 2 TRBD genes ( Fig. 3b ) and all 13 functional TRBJ genes ( Fig. 3c ) were detected in this analysis. As for the TRBV genes, the TRBD and TRBJ genotype and haplotypes were identified on the basis of the alleles identified by IMGT/HighV-QUEST. The individual is heterozygous for TRBD2 (TRBD2*01/TRBD2*02) and TRBJ1-6 (TRBJ1-6*01/TRBJ1-6*02) and homozygous for TRBD1 and the other TRBJ genes (all *01). Thus, the histograms and tables of the IMGT/HighV-QUEST statistical analysis of the TRBV , TRBD and TRBJ gene and allele usage, performed on the ‘1 copy’ ‘single allele’ (for V and J) category, provides an accurate genotype landscape of this individual. Moreover, for the first time, and based on the unambiguous TRBV, TRBD and TRBJ allele determination in V-D-J rearrangements, haplotypes could be described for NGS data. Thus, we demonstrated the respective linkage of the TRBV20-1*01 and TRBJ1-6*01 (and also TRBD2*02) on one chromosome, and of the TRBV20-1*02 and TRBJ1-6*02 (and also TRBD2*01) on the other. No such linkage could be obtained for the TRBV7-3 alleles because no rearrangement was found to TRBJ1-6. These results on the V, D and J genes and alleles provide important clues for the interpretation of sequences of the ‘1 copy’ ‘several alleles’ (for V and/or J) category. They also represent a crucial step towards the definition and characterization of IMGT clonotypes for an accurate description of repertoire immunoprofiles, as described below. IMGT clonotype definition and characterization In the literature, clonotypes are defined differently, depending on the experiment design (functional specificity) or available data. Thus, a clonotype may denote either a complete receptor (e.g., TR alpha - beta), or only one of the two chains of the receptor (e.g., TRA or TRB), or one domain (e.g., V-BETA), or the CDR3 sequence of a domain. Moreover the sequence can be at the amino acid (AA) or nucleotide level, and this is rarely specified. Therefore, our priority was to define clonotypes and their properties, which could be identified and characterized by IMGT/HighV-QUEST, unambiguously. In IMGT, the clonotype, designated as ‘IMGT clonotype (AA)’, is defined by a unique V-(D)-J rearrangement (with IMGT gene and allele names determined by IMGT/HighV-QUEST at the nucleotide level [21] , [22] , [23] , [24] , [25] ) and a unique CDR3-IMGT AA (in-frame) junction sequence [39] , [40] , [41] . To identify ‘IMGT clonotypes (AA)’ in a given IMGT/HighV-QUEST data set, the ‘1 copy’ are filtered to select for sequences with in-frame junction, conserved anchors 104 and 118 ‘C, F’ (‘C’ is 2nd-CYS 104, and ‘F’ is the J-PHE 118 of V-BETA) [36] , [37] , [38] and for V and J functional or ORF, and ‘single allele’ (for V and J; Supplementary Fig. S1 ). By definition, an ‘IMGT clonotype (AA)’ is ‘unique’ for a given data set ( Fig. 4a ). Consequently, each ‘IMGT clonotype (AA)’, in a given data set, has a unique set identifier (column ‘Exp. ID’) and, importantly, has a unique representative sequence (link in column ‘Sequence ID’) selected by IMGT/HighV-QUEST among the ‘1 copy’ ‘single allele’ (for V and J), based on the highest per cent of identity of the V-REGION (‘V %’) compared with that of the closest germline, and/or on the sequence length (thus, the most complete V-REGION). Thus in Fig. 4a , the ‘IMGT clonotype (AA)’ #17081, with an Exp. ID ‘13915-MIDAB_all’, has a unique rearrangement ‘TRBV20-1*02F – TRBD1*01F – TRBJ1-1*01F’, with a CDR3-IMGT length (AA) of ‘12 AA’ and a CDR3-IMGT sequence (AA) ‘SAPAEGGNTEAF’, and conserved anchors 104 and 118 ‘C, F’ (recall of the filter). The IMGT clonotype (AA) representative sequence has a V-REGION, which is 100% identical to that of TRBV20-1*02 and a length of 479 nt. 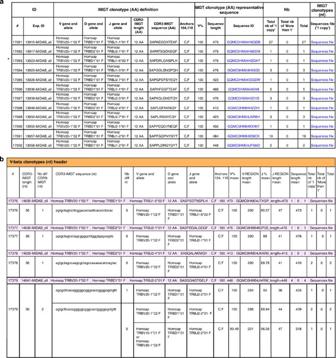Figure 4: IMGT clonotype (AA) and (nt) characterization. This figure represents screenshots from IMGT/HighV-QUEST online. (a) IMGT clonotypes (AA). ‘Exp. ID’ is the identifier of the ‘IMGT clonotype (AA)’ in the data set. The IMGT clonotype (AA) definition includes the names of the V, D, J genes and alleles, the CDR3-IMGT length (AA), the CDR3-IMGT sequence (AA) and the anchors 104 and 118 of the junction ‘C, F’ (for 2nd-CYS 104 and J-PHE F118 for V-BETA, respectively). ‘V%’ indicates the percentage identity of the V-REGION of the representative sequence with the closest germline V-REGION, the sequence length in nucleotides is provided and a link gives access to the sequence in FASTA format; 'nb' indicates the number of sequences '1 copy' and 'More than 1' assigned to the clonotype, and the total. In the ‘IMGT clonotypes (nt)’ column, ‘Sequences file’ gives access to a file containing the '1 copy' sequences assigned to a given IMGT clonotype (AA), in FASTA format. An asterisk (#17083) indicates an example of IMGT clonotype (AA) with a TRBV20-1*02-TRBD1*01-TRBJ1-6*02 rearrangement as described in the genotype and haplotype identification. This figure shows a very small part of the list of the 22,234 unique IMGT clonotypes (AA) identified in this case study. (b) IMGT clonotypes (nt). The nb of different CDR3-IMGT (nt) indicates the nb of IMGT clonotypes (nt) for a given IMGT clonotype (AA) (for example, 2 for #17379). The CDR3-IMGT sequence (nt) is shown with the nb of different nt (nb diff nt). ‘0’ indicates that the CDR3-IMGT (nt) is identical to that of the IMGT clonotype (AA) representative sequence. For #17379, there is an IMGT clonotype (nt) with 1 nt difference (‘c’ instead of ‘t’ at the third position, compared with the CDR3-IMGT of the representative sequence). #17379 also shows an example of ‘several alleles’ (for V and J) assigned to an IMGT clonotype (AA). Figure 4: IMGT clonotype (AA) and (nt) characterization. This figure represents screenshots from IMGT/HighV-QUEST online. ( a ) IMGT clonotypes (AA). ‘Exp. ID’ is the identifier of the ‘IMGT clonotype (AA)’ in the data set. The IMGT clonotype (AA) definition includes the names of the V, D, J genes and alleles, the CDR3-IMGT length (AA), the CDR3-IMGT sequence (AA) and the anchors 104 and 118 of the junction ‘C, F’ (for 2nd-CYS 104 and J-PHE F118 for V-BETA, respectively). ‘V%’ indicates the percentage identity of the V-REGION of the representative sequence with the closest germline V-REGION, the sequence length in nucleotides is provided and a link gives access to the sequence in FASTA format; 'nb' indicates the number of sequences '1 copy' and 'More than 1' assigned to the clonotype, and the total. In the ‘IMGT clonotypes (nt)’ column, ‘Sequences file’ gives access to a file containing the '1 copy' sequences assigned to a given IMGT clonotype (AA), in FASTA format. An asterisk (#17083) indicates an example of IMGT clonotype (AA) with a TRBV20-1*02-TRBD1*01-TRBJ1-6*02 rearrangement as described in the genotype and haplotype identification. This figure shows a very small part of the list of the 22,234 unique IMGT clonotypes (AA) identified in this case study. ( b ) IMGT clonotypes (nt). The nb of different CDR3-IMGT (nt) indicates the nb of IMGT clonotypes (nt) for a given IMGT clonotype (AA) (for example, 2 for #17379). The CDR3-IMGT sequence (nt) is shown with the nb of different nt (nb diff nt). ‘0’ indicates that the CDR3-IMGT (nt) is identical to that of the IMGT clonotype (AA) representative sequence. For #17379, there is an IMGT clonotype (nt) with 1 nt difference (‘c’ instead of ‘t’ at the third position, compared with the CDR3-IMGT of the representative sequence). #17379 also shows an example of ‘several alleles’ (for V and J) assigned to an IMGT clonotype (AA). Full size image Clonal diversity and clonal expression In this study, 22,234 unique IMGT clonotypes (AA) were identified and a representative sequence was assigned to each ( Supplementary Fig. S1 ). The ‘1 copy’ ‘single allele’ sequences not selected as representative (25,153 sequences) were each then assigned to a characterized IMGT clonotype (AA). These sequences differ from the representative sequence by a different (usually shorter) length, and/or by sequencing errors in the V-REGION (lower ‘V %’ of identity) or in the J-REGION, and/or by nucleotide differences in the CDR3-IMGT. These sequences with nucleotide differences in the CDR3-IMGT are identified as ‘IMGT clonotypes (nt)’. The nucleotide differences may be due to sequencing errors or, if this can be proven experimentally, molecular convergence. A given ‘IMGT clonotype (AA)’ may have one or several ‘IMGT clonotypes (nt)’. Thus in Fig. 4b , the ‘IMGT clonotype (AA)’ #17379 has two ‘IMGT clonotypes (nt)’, as shown by the number (‘2’) of different CDR3-IMGT sequences (nt) (‘Nb diff CDR3-IMGT (nt)’). The ‘1 copy’ ‘several alleles (or genes)’ sequences are also assigned to an ‘IMGT clonotype (AA)’, provided that they have the same CDR3-IMGT (AA) and the same V and J alleles of the representative ‘IMGT clonotype (AA)’ among those proposed by IMGT/HighV-QUEST ( Fig. 4b ). In our study, 2,052 ‘several alleles (or genes)’ sequences could be assigned to an ‘IMGT clonotype (AA)’ ( Supplementary Fig. S1 ). The nb of sequences of ‘More than 1’ for each ‘1 copy’ assigned to an IMGT clonotype (AA) is finally included (795 sequences). Thus, by proceeding stepwise to assign sequences, the high quality and specific characterization of the ‘IMGT clonotype (AA)’ remain unaltered. For the first time, for NGS antigen receptor data analysis, our standardized approach allows a clear distinction and accurate evaluation between clonal diversity (nb of ‘IMGT clonotypes (AA)’) and clonal expression (nb of sequences assigned, unambiguously, to a given ‘IMGT clonotype (AA)’). In our study, the 22,234 ‘IMGT clonotype (AA)’ (clonal diversity) corresponded to 50,234 sequences (clonal expression), which represented 78.2% of the filtered-in sequences ( Supplementary Fig. S1 ). These assignments are clearly described and visualized in detail, so the user can check clonotypes, individually. Indeed, the sequences of each ‘1 copy’ assigned to a given ‘IMGT clonotype (AA)’ are available in ‘Sequences file’ ( Fig. 4a,b ). The user can easily perform an analysis of these sequences online with IMGT/V-QUEST (up to 50 sequences, selecting ‘Synthesis view display’ and the option ‘Search for insertions and deletions’) and/or with IMGT/JunctionAnalysis (up to 5,000 junction sequences), which provide a visual representation familiar to the IMGT users. Homo sapiens TRB normalized reference immunoprofiles The comparison of clonal diversity and expression results between studies and experiments requires standards and as these do not exist for NGS, we established Homo sapiens TRB normalized reference immunoprofiles. For clonal diversity, immunoprofiles were obtained by normalizing, to a total of 10,000 clonotypes, the nb of IMGT clonotypes (AA) per TRB (V, D and J) gene (in pink), from the values of 22,231 IMGT clonotypes (AA) (having excluded three abnormal clonotypes, each one represented by a unique sequence) ( Fig. 5 ). For clonal expression, immunoprofiles were obtained by normalizing to a total of 10,000 sequences, the nb of sequences assigned to IMGT clonotypes (AA) per TRBV (in green), TRBD (in red) and TRBJ (in yellow) gene, from the values of the 50,231 assigned sequences per gene ( Fig. 6 ). Normalized values for clonal diversity and expression are reported for TRBV ( Supplementary Table S3 ), TRBD ( Supplementary Table S4 ) and TRBJ ( Supplementary Table S5 ). These TRB normalized reference immunoprofiles will be used to identify variations of interest between the 12 sets (in preparation), despite the overall similarity of the results obtained for the individual sets (an observation that led us to build the normalized reference from the results of the pooled sets). Similarly, the nb of IMGT clonotypes (AA) per CDR3-IMGT length ( Fig. 7a ) and the nb of sequences assigned to the IMGT clonotypes (AA) per CDR3-IMGT length ( Fig. 7b ) were normalized for 10,000 clonotypes (from 22,231 clonotypes) and for 10,000 sequences (from 50,231 sequences), respectively ( Supplementary Table S6 ). This normalized distribution of clonotypes and sequences per CDR3-IMGT length will be used for comparison between the different sets (in preparation) or for results comparison with other studies performed with the same IMGT/HighV-QUEST standards. 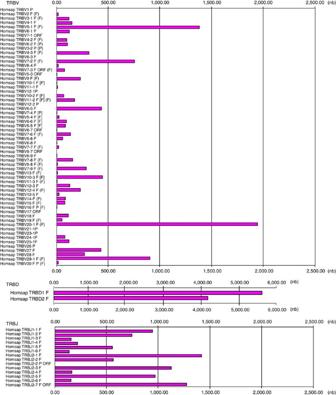Figure 5: Normalized histogram forHomo sapiensTRB clonal diversity. Histograms represent the nb of IMGT clonotypes (AA) per V, D and J genes (in pink) (clonal diversity). Values for clonal diversity (nb of IMGT clonotypes (AA) per V, D and J genes) were normalized for 10,000 IMGT clonotypes (AA). This normalized TRB clonal diversity repertoire was derived from a single individual and had no detectable bias. It represents a TRB immunoprofile reference for comparative analysis of TR V-BETA clonal diversity per V, D and J genes in studies performed with the same IMGT/HighV-QUEST standards. Figure 5: Normalized histogram for Homo sapiens TRB clonal diversity. Histograms represent the nb of IMGT clonotypes (AA) per V, D and J genes (in pink) (clonal diversity). Values for clonal diversity (nb of IMGT clonotypes (AA) per V, D and J genes) were normalized for 10,000 IMGT clonotypes (AA). This normalized TRB clonal diversity repertoire was derived from a single individual and had no detectable bias. It represents a TRB immunoprofile reference for comparative analysis of TR V-BETA clonal diversity per V, D and J genes in studies performed with the same IMGT/HighV-QUEST standards. 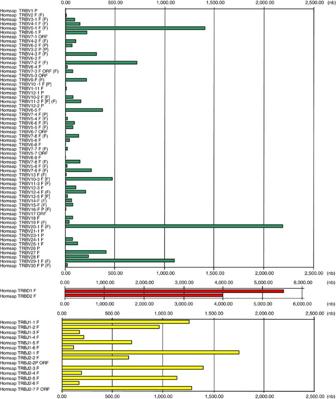Figure 6: Normalized histogram forHomo sapiensTRB clonal expression. Histograms represent the nb of sequences assigned to IMGT clonotypes (AA) per V (in green), D (in red) and J (in yellow) genes (clonal expression). Values for clonal expression (nb of sequences assigned to IMGT clonotypes (AA) per V, D and J genes) were normalized for 10,000 sequences assigned to IMGT clonotypes (AA). This normalized TRB clonal expression repertoire was derived from a single individual and had no detectable bias. It represents a TRB immunoprofile reference for comparative analysis of TR V-BETA clonal expression per V, D and J genes in studies performed with the same IMGT/HighV-QUEST standards. Full size image Figure 6: Normalized histogram for Homo sapiens TRB clonal expression. Histograms represent the nb of sequences assigned to IMGT clonotypes (AA) per V (in green), D (in red) and J (in yellow) genes (clonal expression). Values for clonal expression (nb of sequences assigned to IMGT clonotypes (AA) per V, D and J genes) were normalized for 10,000 sequences assigned to IMGT clonotypes (AA). This normalized TRB clonal expression repertoire was derived from a single individual and had no detectable bias. It represents a TRB immunoprofile reference for comparative analysis of TR V-BETA clonal expression per V, D and J genes in studies performed with the same IMGT/HighV-QUEST standards. 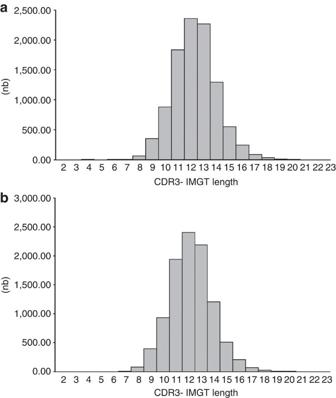Figure 7: Normalized histogram forHomo sapiensTRB CDR3-IMGT length. (a) The histogram represents the nb of IMGT clonotypes (AA) per CDR3-IMGT length. Values for clonal diversity (nb of IMGT clonotypes (AA) per CDR3-IMGT length) were normalized for 10,000 IMGT clonotypes (AA). (b) The histogram represents the nb of sequences assigned to IMGT clonotypes (AA) per CDR3-IMGT length. Values for clonal expression (nb of sequences assigned to IMGT clonotypes (AA) per CDR3-IMGT length) were normalized for 10,000 sequences assigned to IMGT clonotypes (AA). These TRB clonal diversity and expression repertoires per CDR3-IMGT length were from a single individual and had no detectable bias. They represent TRB immunoprofile references for comparative analysis of TR V-BETA clonal diversity and expression repertoires per CDR3-IMGT length in studies performed with the same IMGT/HighV-QUEST standards. Full size image Figure 7: Normalized histogram for Homo sapiens TRB CDR3-IMGT length. ( a ) The histogram represents the nb of IMGT clonotypes (AA) per CDR3-IMGT length. Values for clonal diversity (nb of IMGT clonotypes (AA) per CDR3-IMGT length) were normalized for 10,000 IMGT clonotypes (AA). ( b ) The histogram represents the nb of sequences assigned to IMGT clonotypes (AA) per CDR3-IMGT length. Values for clonal expression (nb of sequences assigned to IMGT clonotypes (AA) per CDR3-IMGT length) were normalized for 10,000 sequences assigned to IMGT clonotypes (AA). These TRB clonal diversity and expression repertoires per CDR3-IMGT length were from a single individual and had no detectable bias. They represent TRB immunoprofile references for comparative analysis of TR V-BETA clonal diversity and expression repertoires per CDR3-IMGT length in studies performed with the same IMGT/HighV-QUEST standards. Full size image IMGT clonotypes (AA) in different T cell subpopulations Analysing an immune response implies the ability to identify the emergence of new IMGT clonotypes (AA) and track memory clonotypes within T cell subpopulations. Whereas the overall immunoprofile was similar between the 12 sets as indicated above, this contrasted with the high diversity of the ‘IMGT clonotypes (AA)’ sequences. Of the total of 22,231 IMGT clonotypes (AA) (50,231 sequences), 21,164 (40,898 seq) were unique to a set, with the following T cell subpopulation distribution: 6,234 clonotypes (12,854 seq) unique to CD4 − sets, 9,492 (16,074 seq) to CD4 + sets and 5,438 (11,970 seq) to Treg sets. In contrast, 1,067 IMGT clonotypes (AA) were common to 2–7 sets (9,237 seq). Among these, 825 (6,525 seq) were common only to sets of the same T cell subpopulation, whereas 242 (2,712 seq) were common to sets between different T cell subpopulations, underlying the importance of studying clonotypes at the sequence level. The low number of common clonotypes between different T cell subpopulations at any given time point confirmed that the flow cytometry separation was effective. Only two IMGT clonotypes (AA) were found in seven sets and were the only common clonotypes pre-vaccination in the three T cell subpopulations. Common ‘IMGT clonotypes (AA)’ were identified post-vaccination, either within a given T cell subpopulation between different time points d3, d8 and d26 (28 clonotypes (272 seq), of which 8 (95 seq) were in CD4 − sets, 4 (36 seq) in CD4 + sets and 16 (141 seq) in Treg sets), or between two T cell subpopulations (9 clonotypes (63 seq)), but no common clonotypes could be identified between all three T cell subpopulations at any time point post-vaccination. The clonotypes emerging after vaccination required more extensive molecular characterization and analysis. This however is associated with biological analysis, and beyond the scope of this study. Therefore, we focused on the IMGT clonotypes (AA), common at the four time points within a given T cell subpopulation. Thus, 82 IMGT clonotypes (AA), namely 29, 11 and 42 in the CD4 − , CD4 + and Treg sets, respectively, were identified and followed individually. These IMGT clonotypes (AA) used different TRBV genes and alleles ( Fig. 8 ). Whereas the TRBV gene and allele distribution differed between the three T cell subpopulations, the pattern was strikingly similar within a subpopulation at different time points. This supports the reproducibility of the IMGT/HighV-QUEST determination of the IMGT clonotypes (AA), between experiments, and importantly, means that if variability was observed (for example, in the case of CD4 + in Fig. 8 ), this warrants exploration for either experimental bias or biological significance. The individual clonal expression of the 82 common IMGT clonotypes (AA) within a given T cell subpopulation could also be followed using the IMGT/HighV-QUEST statistical analysis results, based on the nb of sequences assigned to each at the four time points and normalized for 10,000 sequences, in the CD4 − sets ( Supplementary Fig. S2a ), CD4 + sets ( Supplementary Fig. S2b ) and Treg sets ( Supplementary Fig. S2c ). 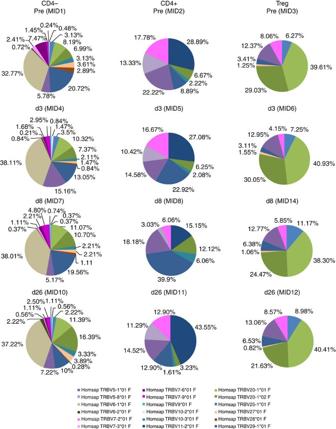Figure 8:TRBVgenes and alleles in common IMGT clonotypes (AA). As a control of the feasibility of following IMGT clonotypes (AA) common to different sets, the distribution of theTRBVgenes and alleles was taken as an indicator. The 82 IMGT clonotypes (AA) that were common at the four time points within a given T cell subpopulation were selected (29 in the CD4−sets, 11 in the CD4+sets and 42 in the Treg sets). The percentage of the nb of sequences assigned to the IMGT clonotypes (AA) and characterized by theirTRBVgene and allele, normalized for 10,000 sequences, is graphically represented with four pie graphs for the four time points (pre-vaccination (Pre), post-vaccination at day 3 (d3), day 8 (d8) and day 26 (d26)), displayed vertically per T cell subpopulation (CD4−, CD4+, Treg). Figure 8: TRBV genes and alleles in common IMGT clonotypes (AA). As a control of the feasibility of following IMGT clonotypes (AA) common to different sets, the distribution of the TRBV genes and alleles was taken as an indicator. The 82 IMGT clonotypes (AA) that were common at the four time points within a given T cell subpopulation were selected (29 in the CD4 − sets, 11 in the CD4 + sets and 42 in the Treg sets). The percentage of the nb of sequences assigned to the IMGT clonotypes (AA) and characterized by their TRBV gene and allele, normalized for 10,000 sequences, is graphically represented with four pie graphs for the four time points (pre-vaccination (Pre), post-vaccination at day 3 (d3), day 8 (d8) and day 26 (d26)), displayed vertically per T cell subpopulation (CD4 − , CD4 + , Treg). Full size image Although NGS exhibits great potential for the analysis of the immune repertoire, NGS data per se are still heavily biased owing to experimental and methodological flaws from the sample preparation, to TR transcript amplification, or to the sequencing and interpretation of the results. In this study, we used a combination of 5′RACE, 454 and IMGT/HighV-QUEST for standardized analysis of complete V domains, for genotype/haplotype analysis, characterization of IMGT clonotypes (AA), clonal diversity and clonal expression, and generation of immune profiles in normal repertoires and during disease. The 5′RACE [12] , [26] is reliable for TR repertoire analysis as shown by the overall consistency of the clonotypic and expression histograms of 12 different sets (corresponding to three T cell subpopulations at four time points) and confirmed by the detection of rearranged transcripts of in-frame pseudogenes (which may be used as internal controls). Whereas the 5′RACE PCR introduced few errors, probably due to the use of high-fidelity polymerases and low cycle numbers, recent studies established that the majority of errors in TR deep sequencing occur during the solid-phase steps [42] . Interestingly, IMGT/HighV-QUEST analysis detects and corrects insertions and/or deletions, which represent current sequencing errors found with 454 due to homopolymer hybridization. The IMGT/HighV-QUEST functionality ‘Search for insertions and deletions’ is provided by default owing to the high number of indels observed in NGS data. This functionality is identical to that created in IMGT/V-QUEST [22] , [25] online, as an option for analysis of sequences from leukaemic cells in which indels are frequent [23] . Sequencing errors in the CDR3-IMGT are not corrected by IMGT/HighV-QUEST, however our characterization of ‘IMGT clonotypes (nt)’ highlights sequences with CDR3-IMGT nt differences for each IMGT clonotype (AA). With free public online access, IMGT/HighV-QUEST allows our approach to be readily adaptable to other studies. IMGT/HighV-QUEST analyses directly the fully rearranged IG and TR V-J and V-D-J sequences, without the need of computational assembly. IMGT/HighV-QUEST is a generic tool that allows analysis of IG and TR of different species, including identification of new allele IG and TR polymorphisms and analysis of IG somatic hypermutations. Therefore, IMGT/HighV-QUEST requires NGS methodology, which provides sufficiently long and reliable sequences encompassing directly the V domain. The current average read length of 454 sequencing is ~400 nt (431 nt for the ‘1 copy’ in this study). A major feature of our work was to define and characterize ‘IMGT clonotype (AA)’ to determine their nb (clonal diversity) and to identify the nb of sequences assigned to each ‘IMGT clonotype (AA)’ (clonal expression). This requires several steps in the IMGT/HighV-QUEST statistical analysis. First, IMGT clonotypes (AA) are identified among the ‘1 copy’ with in-frame junctions, conserved anchors 104 and 118 (‘C, F’ for 2nd-CYS and V-BETA J-PHE, respectively), V and J functional or ORF, ‘single allele’ (for V and J). Their characterization includes the identification of the rearranged TRBV and TRBJ gene and allele at the nucleotide level by IMGT/HighV-QUEST, and that of a unique CDR3-IMGT (AA) sequence. As a given clonotype may be identified in sequences that differ in length and/or contain sequencing errors, a representative sequence (highest percentage identity of the V-REGION and longest sequence) and an identifier are assigned to each IMGT clonotype (AA) identified in a given data set. Second, the nb of sequences for an IMGT clonotype (AA) (clonal expression) is obtained by aggregating to the representative sequence the nb of sequences that are not selected as representative. The ‘Sequences file’ of the IMGT clonotypes (AA) allows a comparison of all the sequences assigned to a given clonotype (AA). We demonstrate that common IMGT clonotypes (AA) can be followed at different time points between T cell subpopulations, revealing the feasibility of a standardized approach for analysis of specific clones in the immune response. As a large number of antigens are implicated in any infection, it is impossible to identify and simultaneously investigate all antigen-specific T cells mobilized against a complex pathogen. IMGT/HighV-QUEST is capable of quantitatively analysing almost half a million (450,000) results of sequences, simultaneously. With more than 530 columns of results per sequence ( Supplementary Table S7 ), the nb of data analysed is >2 × 10 8 , and represents a genuine advance in standardized and high-quality TR repertoire analysis. It is becoming increasingly apparent that the nature of the T cell repertoire deployed during an immune response can directly affect disease outcomes [7] , [9] , [43] , [44] , [45] , [46] . As such, new tools and a standardized methodology (as presented in this case study) capable of dissecting the TR repertoire in a rapid, detailed and comprehensive fashion will be helpful in uncovering new immunopathological associations and accelerate knowledge of basic TR repertoire biology. Presently, TR repertoire investigation is limited by two polarizing challenges. At one end, high-throughput sequencing alone cannot correlate a clonotype with its functional parameters. At the other end, Sanger sequencing of sorted cells has low throughput and the method depends on prior knowledge of the antigen and/or the antigen-specific cells, thus often missing many antigen-specific populations. Combining high-throughput TR immunoprofiling using IMGT/HighV-QUEST analysis with cell identity-oriented approaches will bring genuine advances in TR repertoire studies in health and disease. Ethics statement The study was approved by the Alfred Hospital Research Ethics Committee and the Victorian Department of Human Services Human Research Ethics Committee. Written informed consent was obtained from the volunteer. Cells and RNA A 45-year-old healthy male Caucasoid volunteer (HLA- A*0201/*3002, B*1501/*1801, C*0303/*0501, DRB1*0301/*0401, DQB1*0302/*0201) was vaccinated with H1N1 vaccine (Panvax H1N1 Vaccine, CSL), and blood samples were collected before vaccination and on days 3, 8 and 26 post-vaccination. PBMC at each time point were depleted of CD14 + and CD19 + cells using MACS (Miltenyi Biotec), stained for CD4, CD3, CD25 and CD127 surface expression (fluorochrome-conjugated monoclonal antibodies from BD Biosciences) and then sorted into three T cell subpopulations: regulatory T cells (‘Treg’, with a phenotype CD3 + CD25 + CD127 −/lo ) [27] and conventional T cells CD3 + CD4 + (‘CD4 +’ ) and CD3 + CD4 − (‘CD4 − ’) using FACSAria (BD Biosciences) ( Fig. 1a ). Treg cells [27] , [28] , [29] , [30] , which represent a minor subpopulation (~5% ) within circulating T cells (or ~2% of PBMC) were included in the analysis to evaluate if the technique works for both abundant T cell subpopulations (e.g., CD4 + ) as well as small subpopulations. RNA was immediately extracted from sorted cells using RNeasy minikit (Qiagen). In one experiment, DNA was extracted from CD14 + and CD19 + cells, and was subsequently used in high-resolution HLA class I and II typing [29] . Amplicon library construction The concentration of RNA was determined using a NanoDrop ND-8000 spectrophotometer and ~200 ng RNA was used for each library. TRB transcripts were amplified using 5′RACE PCR [12] , [26] because this strategy provides an unbiased amplification of full, rearranged V-D-J sequences. We chose to amplify mRNA over rearranged genomic DNA to obtain sufficiently long sequences with complete V domains, by avoiding the intervening sequence between J and C. A total of 12 libraries were constructed, corresponding to the 12 blood samples (three T cell subpopulations × four time points), using established protocols [12] , [13] with minor modifications. In brief, a 5′RACE PCR was conducted using the SMARTer RACE cDNA Amplification Kit (Clontech Laboratories) according to the manufacturer’s instructions. The extension time for the first-strand cDNA synthesis was 90 min at 42 °C followed by 15-min inactivation at 70 °C. The first-round PCR was achieved using Phusion Hot-Start DNA Polymerase (Finnzymes), a template-switching oligonucleotide (TSO), a universal primer mix (supplied in the above SMARTer RACE cDNA amplification kit), along with the TRBC gene-specific reverse primer, 5′-TTCTGATGGCTCAAACAC-3′ (codon positions 11-6, IMGT unique numbering), which aligns to both TRBC1 and TRBC2 genes [1] , [31] (IMGT Repertoire, http://www.imgt.org ). The cycling conditions were: 30 s denaturation at 98 °C, 26 cycles of 10 s at 98 °C, 10 s at 55 °C and 20 s at 72 °C, plus a final extension for 5 min at 72 °C. The reaction products were purified using QIAquick columns (Qiagen). The purified DNA fragment was loaded on a 1.5% low melting temperature agarose gel, and a band corresponding to a 500- to 650-bp product was excised and purified using the QIAquick Gel Extraction Kit (Qiagen). A second-round PCR was performed on a fraction of the first-round reaction. This step incorporated Roche forward and reverse linker primers to enable the sequencing and the Multiplex Identifier (MID) or barcodes (MID1–MID8, MID10–MID12 and MID14) to distinguish the different cell fractions and time points (454 Sequencing Technical bulletin TCB N°013-2009, August 2009). The product of the second-round PCR was purified as described above, and quantified using PicoGreen reagent (Invitrogen). Finally, an equal amount (100 ng) of cDNA from each of the 12 libraries was pooled to obtain the final amplicon library, which represents the complete collection of TRBV transcripts sampled from this donor ( Fig. 1b ). Sequencing and initial data processing Sequencing was performed on a ¼ PicoTiterPlate by the Australian Genome Research Facility using the 454 Genome Sequencer FLX (GSFLX) Titanium (Roche). Initial data processing was performed using the manufacturer's software, which included the removal of low quality and erroneous sequences as determined by the standard filters of the Roche amplicon signal-processing pipeline. Sequences were assigned to samples based on incorporated barcodes, and read orientation was determined by the presence or absence of the sequence corresponding to the TSO used in the SMARTer RACE. Sequence segments corresponding to the adapters, barcodes and TSO were removed during this process. Quality control was conducted by spiking the amplicon library using classical cloning and sequencing methods [7] , [11] . Repertoire analysis using IMGT/HighV-QUEST The ‘final 454-output’ reads were submitted online to IMGT/HighV-QUEST [21] , [22] . The full capacity of IMGT/HighV-QUEST includes analysis of V-J and V-D-J rearranged sequences (up to 150,000 per job) and statistical analysis (on results of up to 450,000 sequences) ( http://www.imgt.org , version July 2012). The IMGT/HighV-QUEST [21] submission page allows users to submit a file containing up to 150,000 sequences and to select options (equivalent to those of IMGT/V-QUEST [22] , [23] , [24] , [25] ) for the results display. The results are provided in a downloadable main folder with 11 files [21] ( Supplementary Table S7 ) in CSV format (results equivalent to those of the Excel file from IMGT/V-QUEST online [22] , [23] , [24] , [25] ), and one folder with the individual files (up to 150,000) of all the sequence results [21] . For each analysed sequence, the results in those individual files are identical to those that could be obtained from IMGT/V-QUEST online (in display option ‘Text’ of 'Detailed view' [22] , [23] , [24] , [25] ). Text and CSV formats facilitate statistical studies for further interpretation and information extraction. Before IMGT/HighV-QUEST analysis, the users can evaluate the quality of their sequences by checking the results obtained with IMGT/V-QUEST on a few sequences. In a second online step, the users can submit the results of one or several jobs (up to 450,000 results) for statistical analysis. The IMGT/HighV-QUEST ‘Summary’ table of the statistical analysis provides information in Results categories that are either filtered in (‘1 copy’, ‘More than 1’) or filtered out (‘Warnings’, ‘Unknown functionality’, ‘No results’) [21] . The number of sequences in the different categories provides the users with an immediate indication of data reliability. Before the final results, statistical analyses were also performed on ‘MIDA_all’ and ‘MIDB_all’ separately, and on the 5′ reads and 3′ reads separately of each of the 12 samples for the purpose of data evaluation. The 5′ and 3′ reads were pooled to overcome the limitation of 454 sequencing, which does not provide genuine ‘bi-directional’ sequences. Indeed, the 5′ reads and 3′ reads are generated independently in separate wells, and the comparison of the IMGT/HighV-QUEST statistical analysis performed on the 5′ or 3′ reads, separately or pooled, confirmed the necessity of pooling to avoid losing information. Genotype and haplotypes identification The genotype and haplotypes were deduced from the IMGT/HighV-QUEST statistical analysis performed on all pooled sets (‘MIDA+MIDB’) on the results category ‘1 copy’ ‘single allele’ (for V and J). Accession code: Sequencing data has been deposited in the NCBI Sequence Read Archive under accession code SRX326382 . How to cite this article: Li, S. et al . IMGT/HighV QUEST paradigm for T cell receptor IMGT clonotype diversity and next generation repertoire immunoprofiling. Nat. Commun. 4:2333 doi: 10.1038/ncomms3333 (2013).